Structural determinants of HIV-1 Vif susceptibility and DNA binding in APOBEC3F The human APOBEC3 family of DNA cytosine deaminases serves as a front-line intrinsic immune response to inhibit the replication of diverse retroviruses. APOBEC3F and APOBEC3G are the most potent factors against HIV-1. As a countermeasure, HIV-1 viral infectivity factor (Vif) targets APOBEC3s for proteasomal degradation. Here we report the crystal structure of the Vif-binding domain in APOBEC3F and a novel assay to assess Vif-APOBEC3 binding. Our results point to an amphipathic surface that is conserved in APOBEC3s as critical for Vif susceptibility in APOBEC3F. Electrostatic interactions likely mediate Vif binding. Moreover, structure-guided mutagenesis reveals a straight ssDNA-binding groove distinct from the Vif-binding site, and an ‘aromatic switch’ is proposed to explain DNA substrate specificities across the APOBEC3 family. This study opens new lines of inquiry that will further our understanding of APOBEC3-mediated retroviral restriction and provides an accurate template for structure-guided development of inhibitors targeting the APOBEC3-Vif axis. The human intrinsic immune system has developed complex responses to prevent the spread of retroviral pathogens. The apolipoprotein B mRNA-editing catalytic polypeptide-like 3 (APOBEC3, denoted here as A3) [1] , [2] , [3] family of single-stranded (ss) DNA cytosine deaminases provides a critical post-entry obstruction to retroviral replication. In humans, seven family members (A3A, A3B, A3C, A3D, A3F, A3G and A3H) are encoded on chromosome 22 ( Fig. 1a ) [4] . A common characteristic of all A3 enzymes is the presence of either one or two zinc-coordinating, DNA cytosine deaminase domains, typically labelled as CD1 and CD2 (ref. 4 ). Each cytosine deaminase domain contains the canonical (C/H)-(A/V)-E-(X 23-28 )-P-C-X 2 -C motif and belongs to one of three classes: Z1 (A3A and the CD2 of A3B and A3G), Z2 (A3C, the CD1 of A3B and A3G, and both CD1 and CD2 of A3D and A3F) or Z3 (A3H haplotype II) [5] . Z2-cytosine deaminase domains can be further divided into three subgroups: A3F-CD1 (CD1 of A3B, A3D and A3F), A3F-CD2 (A3C, and CD2 of A3D and A3F) and A3G-CD1 subgroups ( Fig. 1a ). 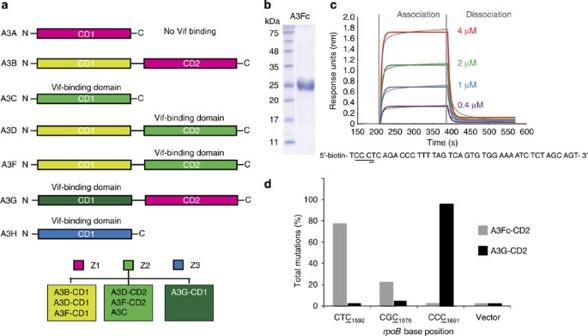Figure 1: APOBEC3 and characterization of A3Fc-CD2. (a) Schematic of the seven A3 intrinsic immune restriction factors (A3A, A3B, A3C, A3D, A3F, A3G and A3H). The three classes of DNA cytosine deaminase domains, Z1, Z2 and Z3 are coloured pink, green and blue, respectively. The Z2-cytosine deaminase domains are further classified into three subgroups based on sequence similarity. A3F and A3G are the two most potent A3 proteins and exhibit disparate Vif-binding sites (CD1 for A3G and CD2 for A3F). (b) SDS–PAGE of the purified A3Fc-CD2 after final size exclusion chromatography. (c) BLI kinetic analysis of A3Fc-CD2 binding to ssDNA. Biotin-labelled ssDNA was coupled to streptavidin-coated biosensors and monitored for binding to purified A3Fc-CD2 at 0, 0.4, 1, 2 and 4 μM concentrations. The data was analysed based on a 1:1 binding model using the BLItz Pro software, with the fitted curves shown as grey lines. The ssDNA sequence used in the assay is shown below the sensorgram, with the A3Fc-CD2 deamination site and target DNA cytosine underlined and double underlined, respectively. (d) RifRmutation profile ofE. coliexpressed A3Fc-CD2 and A3G-CD2. Histogram showing the percent mutation on specificrpoBnucleotide sequences for A3Fc-CD2 and A3G-CD2. Results are expressed as the percentage of total mutations from six independent experiments with at least 20 RifRcolonies sequenced for both A3Fc-CD2 and A3G-CD2. Figure 1: APOBEC3 and characterization of A3Fc-CD2. ( a ) Schematic of the seven A3 intrinsic immune restriction factors (A3A, A3B, A3C, A3D, A3F, A3G and A3H). The three classes of DNA cytosine deaminase domains, Z1, Z2 and Z3 are coloured pink, green and blue, respectively. The Z2-cytosine deaminase domains are further classified into three subgroups based on sequence similarity. A3F and A3G are the two most potent A3 proteins and exhibit disparate Vif-binding sites (CD1 for A3G and CD2 for A3F). ( b ) SDS–PAGE of the purified A3Fc-CD2 after final size exclusion chromatography. ( c ) BLI kinetic analysis of A3Fc-CD2 binding to ssDNA. Biotin-labelled ssDNA was coupled to streptavidin-coated biosensors and monitored for binding to purified A3Fc-CD2 at 0, 0.4, 1, 2 and 4 μM concentrations. The data was analysed based on a 1:1 binding model using the BLItz Pro software, with the fitted curves shown as grey lines. The ssDNA sequence used in the assay is shown below the sensorgram, with the A3Fc-CD2 deamination site and target DNA cytosine underlined and double underlined, respectively. ( d ) Rif R mutation profile of E. coli expressed A3Fc-CD2 and A3G-CD2. Histogram showing the percent mutation on specific rpoB nucleotide sequences for A3Fc-CD2 and A3G-CD2. Results are expressed as the percentage of total mutations from six independent experiments with at least 20 Rif R colonies sequenced for both A3Fc-CD2 and A3G-CD2. Full size image Experiments with cultured cells demonstrate that only A3D, A3F, A3G and A3H restrict HIV-1 (ref. 6 ), and that A3F and A3G are the most abundant and potent inhibitors [7] , [8] , [9] . Both A3F and A3G are double-domain DNA cytosine deaminases, and are expressed and packaged into viral particles as oligomers bound to viral RNA and structural proteins [10] . During reverse transcription, A3 deaminates retroviral DNA cytosines. This conversion of dC to dU results in the incorporation of dA rather than dG in the positive-strand DNA, leading to premature stop codons and detrimental mutations in viral proteins. Of course, HIV-1 has developed countermeasures to antagonize this intrinsic host defence response. HIV-1 viral infectivity factor (Vif) is a late-onset viral protein that recruits an E3 ubiquitin ligase complex (elongin B/C, core binding factor-β, cullin 5, and Rbx-2) to polyubiquitinate A3, leading to its proteasomal degradation and loss of packaging into nascent virions [11] , [12] . In addition, Vif has been shown to impede A3 mRNA translation, virion encapsidation and deamination activity [13] , [14] , [15] . The degradation of A3F and A3G is dependent on recognition and binding of HIV-1 Vif. Interestingly, while A3F and A3G share a high primary sequence similarity of 50.9%, disparate regions in these proteins are involved in binding HIV-1 Vif [16] , [17] . In A3F, the CD2 domain mediates both DNA cytosine deamination and binding to HIV-1 Vif, whereas in A3G, the enzymatically inactive CD1 domain is responsible for binding Vif [18] . Current antiretroviral drug treatments have led to significant improvements in quality of life for those infected with HIV-1 or living with AIDS. However, error-prone HIV-1 replication produces high genetic variation that leads to the natural selection of drug-resistant variants of HIV-1, thus necessitating the development of alternate strategies. The A3F–Vif or A3G–Vif interface is an attractive target as a fresh anti-HIV therapeutic approach [19] . Inhibition of HIV-1 Vif binding to A3F or A3G would allow the reactivation of effective host innate immune responses to HIV-1. More importantly, inhibitors targeting the host side of the A3F–Vif or A3G–Vif interface will be less sensitive to viral mutations and will reduce the probability of HIV-1 variants developing resistance to drug treatments. Here we report the crystal structure of the Vif-binding domain in A3F-CD2. Given that A3F and A3G are the most potent A3 restriction factors, this is a key structure needed for the development of new classes of inhibitors to enhance intrinsic immunity against HIV. We performed site-directed mutagenesis to map out the ssDNA-binding site, which revealed a straight groove for DNA binding, as well as a novel aromatic switch that conferrs nucleotide preferences. Moreover, we developed the first biophysical HIV-1 Vif-APOBEC3 binding assay, and this allowed us to identify a negatively charged Vif-binding surface distinct from the ssDNA-binding groove. A soluble chimeric A3F C-terminal domain A3 family members are difficult to express and purify in soluble, stable and homogeneous quantities. This has hindered structural studies on this important class of macromolecules. Expression of the full-length, CD1 or CD2 A3F domains in Escherichia coli cells resulted in the formation of inclusion bodies. Multiple E. coli cell lines and expression temperatures were tried, but to no avail. Re-engineering of these proteins is necessary to impart solubility and stability. We noticed that residues 195–220 of the A3F-CD2 domain are rich in hydrophobic residues, leading us to hypothesize that these amino acids may lead to protein aggregation. In contrast, residues 197–221 of A3G-CD2 are comparatively less hydrophobic. To generate a soluble construct of A3F-CD2, residues 195–217 of A3F-CD2 were replaced with residues 197–221 from A3G-CD2. This chimeric A3F (A3Fc-CD2) construct ( Supplementary Fig. S1 ) expressed as soluble protein in multi-milligram quantities ( Fig. 1b ). The A3Fc-CD2 was shown by in vitro biochemical and biophysical assays to be fully functional. Using biolayer interferometry (BLI), we found that A3Fc-CD2 binds ssDNA with an equilibrium dissociation constant ( K d ) of 7 μM ( Fig. 1c ), and as expected, does not bind double-stranded DNA. Previous chemical shift perturbation and gel shift assays have shown that A3A and A3G-CD2 bind ssDNA with K d values in the micromolar range [20] , [21] , [22] , consistent with A3Fc-CD2. In addition, a heterologous E. coli DNA cytosine deaminase mutational assay [18] revealed that A3Fc-CD2 was enzymatically active and preferentially targets a 5′-CCTC-3′ sequence in the E. coli RNA polymerase ( rpoB ) gene ( Fig. 1d ), consistent with previous studies that show A3F deamination within 5′-TC-3′ dinucleotide signatures in the rpoB gene [18] . Crystal structure of A3Fc-CD2 A3Fc-CD2 was crystallized using a unique microseeding, discontinuous vapour diffusion method to reduce protein precipitation and improve crystal growth. Diffraction of the crystals presented additional challenges, as most crystals diffracted between 5–10 Å resolution. In the end, only one crystal out of 100 diffracted to ~3.0 Å resolution. The crystal structure of A3Fc-CD2 was determined by molecular replacement and the final refined model consists of A3Fc-CD2 residues 218–373 and a 25-residue N-terminal extension from the corresponding A3G sequence. Data collection and refinement statistics are presented in Table 1 . Table 1 Data collection and refinement statistics. Full size table The crystal structure of A3Fc-CD2 consists of a five-stranded, mixed β-sheet core flanked by three α-helices on either side ( Fig. 2a ). Our overall A3Fc-CD2 structure resembles A3C (PDB: 3VOW) and A3G-CD2 structures (PDB: 3E1U, 2JYW, 2KBO and 3IR2) [21] , [22] , [23] , [24] , [25] . Superimposition of A3Fc-CD2 with A3C and A3G-CD2 revealed an overall Cα root mean-squared deviation of 2.3 Å and 1.3 Å, respectively. The significant resemblance in the overall fold of A3Fc-CD2 to A3G-CD2 and A3C suggests that this is a conserved structural core for the A3 family. 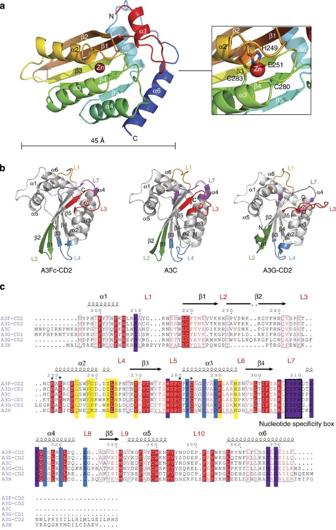Figure 2: Crystal structure of A3Fc-CD2. (a) Ribbon diagram of A3Fc-CD2. The chain is coloured in a rainbow gradient from red (N terminus) to blue (C terminus). The catalytic zinc atom is labelled and shown as a grey sphere. The inset box shows a zoomed view of the catalytic site. (b) Structural difference between A3Fc-CD2, A3G-CD2 and A3C. All APOBEC3 cytosine deaminase domains have 10 loops. The largest structural deviations reside in loops L1, L2, L3, L4 and L7, coloured orange, green, red, blue and purple, respectively. (c) Multiple sequence alignment of A3F-CD2, A3C, A3D-CD2, A3G-CD1, A3G-CD2 and A3H. Numbering of the sequences and depiction of secondary structural elements are based on A3Fc-CD2, and is shown above the sequences. Strictly conserved residues are highlighted in red. Putative A3Fc-CD2 ssDNA-binding and Vif-binding residues are outlined in purple and blue boxes, respectively. Previously identified residues in the hydrophobic V-shaped groove formed by the α2 and α3 helices are outlined in yellow. Catalytic site residues are denoted with an asterisk above its sequence. The sequence alignment was produced using Clustal W51,52and the alignment graphics were generated using the programme ESPript53. Figure 2: Crystal structure of A3Fc-CD2. ( a ) Ribbon diagram of A3Fc-CD2. The chain is coloured in a rainbow gradient from red (N terminus) to blue (C terminus). The catalytic zinc atom is labelled and shown as a grey sphere. The inset box shows a zoomed view of the catalytic site. ( b ) Structural difference between A3Fc-CD2, A3G-CD2 and A3C. All APOBEC3 cytosine deaminase domains have 10 loops. The largest structural deviations reside in loops L1, L2, L3, L4 and L7, coloured orange, green, red, blue and purple, respectively. ( c ) Multiple sequence alignment of A3F-CD2, A3C, A3D-CD2, A3G-CD1, A3G-CD2 and A3H. Numbering of the sequences and depiction of secondary structural elements are based on A3Fc-CD2, and is shown above the sequences. Strictly conserved residues are highlighted in red. Putative A3Fc-CD2 ssDNA-binding and Vif-binding residues are outlined in purple and blue boxes, respectively. Previously identified residues in the hydrophobic V-shaped groove formed by the α2 and α3 helices are outlined in yellow. Catalytic site residues are denoted with an asterisk above its sequence. The sequence alignment was produced using Clustal W [51] , [52] and the alignment graphics were generated using the programme ESPript [53] . Full size image In A3Fc-CD2, the catalytic zinc atom is sequestered by H249, C280 and C283 within the canonical (C/H)-(A/V)-E-(X 23–28 )-P-C-X 2 -C cytidine deaminase motif ( Fig. 2a ). The active site residues superimpose well in all A3 structures. In A3G-CD2 and A3C, a water molecule is coordinated to the catalytic zinc to complete a tetrahedral geometry. This water molecule is activated to become a nucleophile for deamination of the target deoxycytidine nucleotide. In A3Fc-CD2, the catalytic water molecule is not observed due to the moderate resolution of the electron density map. While the overall structure and active site are similar among all A3 proteins, significant differences are observed in the loops that surround the structural core. Loops have higher conformational flexibility than secondary structural elements, and are often involved in crystal packing interactions. All 10 A3Fc-CD2 loops that surround the α/β core superimpose well with those from A3C, suggesting that any loops involved in forming the crystal lattice are not significantly affected. In contrast, superimposition of A3Fc-CD2 and A3C to A3G-CD2 revealed structural differences in loops 1, 2, 3, 4 and 7, with the largest displacements in loops 2 and 3 ( Fig. 2b ). Loop 2 resides between the β1 and β2 strands. The β2 strand in A3Fc-CD2 and A3C forms a 12-residue continuous strand, whereas in A3G-CD2, a bulge disrupts β2 into two four-residue strands (referred to β2 and β2′). Previous NMR and crystallographic experiments showed that the bulge is not an experimental artifact, but rather an intrinsic feature of A3G-CD2 (ref. 25 ). The β2 strand of CD1 was proposed in modeling studies to pair with the β2 strand of CD2 to form an extended β-sheet in full-length A3 structures [26] , [27] , [28] . If this were the case, differences in β2 would likely result in disparities at the intermolecular interface between the two catalytic domains of A3F and A3G. However, recent studies have contradicted this model [24] , [29] and further studies are required to characterize the interface between CD1 and CD2. Loop 3 is formed between the β2 strand and the α2 helix, and a four-residue insertion in loop 3 of A3G-CD2 produces an extended structure compared to A3C and A3Fc-CD2. In A3G, loop 3 may be involved in Zn-mediated oligomerization [25] , whereas in A3Fc-CD2 and A3C, loop 3 is shorter and no such protein–protein interactions were detected. ssDNA-binding site of A3Fc-CD2 In A3Fc-CD2, the molecular surface reveals a single, partial groove that leads into the catalytic site. This groove is formed between loops 1 and 3 on one side and loop 7 on the opposite side. A number of aromatic (W277, Y307, Y308, F309, W310 and Y314), and charged residues (K209, R305, and D313) line the channel ( Fig. 3a,b ). The positively charged R305 and aromatic W277 and Y307 residues are conserved between A3F-CD2 and A3G-CD2, suggesting a key role in ssDNA binding ( Fig. 2c ). Based on the overall active site structure, W277 and Y307 are in close proximity to the catalytic residues and zinc atom ( Fig. 3b ). These two residues are in excellent position to form stabilizing pi–pi interactions to the target nucleotide base. Residue R305 is located directly behind W277 in the active site and forms pi–cation interactions capable of stabilizing W277. Residues Y308, F309, W310 and Y314 line one face of the ssDNA-binding groove and may form base-stacking interactions with other bases on the nucleotide chain (for example, the −1 and −2 positions of the 5′- TT CA-3′ A3F deamination motif). 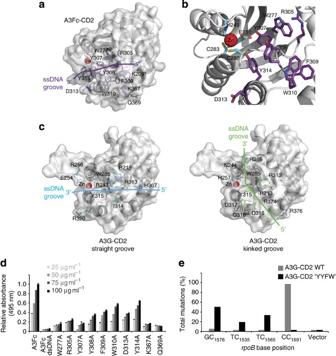Figure 3: Identification of the A3Fc-CD2 ssDNA-binding site. (a) Molecular surface of the putative A3Fc-CD2 ssDNA-binding site. Key residues proposed for DNA binding are shown in purple. Aromatic and positively charges residues line the wall of a straight groove. This DNA binding groove is consistent with Model no. 1 in panel (c). Note: residue W209 belongs to the A3G solubilization linker attached at the N terminus of A3Fc-CD2. The native residue in A3Fc-CD2 is a lysine, and this residue is in position to accommodate the negative charges from the phosphate backbone of the ssDNA strand. (b) A3Fc-CD2 active site. Catalytic and ssDNA-binding residues are shown in cyan and purple sticks, respectively. (c) Two models of A3G-CD2 ssDNA binding. Model no. 1 is proposed by Furukawaet al.22and Chenet al.21and is based on a NMR titration analysis of ssDNA. DNA-binding residues were found to line a straight DNA binding groove. Model no. 2 is proposed by Holdenet al.23and displays the DNA binding residues along a kinked groove. Both A3G-CD2 molecular surfaces are shown in the same orientation as panel (a). (d) Nucleic acid–protein interaction ELISA assay. Alanine scanning mutagenesis of selected A3Fc-CD2 ssDNA-binding site residues. dsDNA was used as a negative control. Results are expressed as the mean relative absorbance (+s.d. of the population) of three replicates. (e) RifRmutation profile ofE. coliexpressed WT A3G-CD2 and A3G-CD2 ‘YYFW’. Histogram showing the percent total mutation on specificrpoBnucleotide sequences. Results are expressed as the percentage of total mutations from six independent experiments with at least 20 colonies sequenced. Figure 3: Identification of the A3Fc-CD2 ssDNA-binding site. ( a ) Molecular surface of the putative A3Fc-CD2 ssDNA-binding site. Key residues proposed for DNA binding are shown in purple. Aromatic and positively charges residues line the wall of a straight groove. This DNA binding groove is consistent with Model no. 1 in panel (c). Note: residue W209 belongs to the A3G solubilization linker attached at the N terminus of A3Fc-CD2. The native residue in A3Fc-CD2 is a lysine, and this residue is in position to accommodate the negative charges from the phosphate backbone of the ssDNA strand. ( b ) A3Fc-CD2 active site. Catalytic and ssDNA-binding residues are shown in cyan and purple sticks, respectively. ( c ) Two models of A3G-CD2 ssDNA binding. Model no. 1 is proposed by Furukawa et al . [22] and Chen et al . [21] and is based on a NMR titration analysis of ssDNA. DNA-binding residues were found to line a straight DNA binding groove. Model no. 2 is proposed by Holden et al . [23] and displays the DNA binding residues along a kinked groove. Both A3G-CD2 molecular surfaces are shown in the same orientation as panel (a). ( d ) Nucleic acid–protein interaction ELISA assay. Alanine scanning mutagenesis of selected A3Fc-CD2 ssDNA-binding site residues. dsDNA was used as a negative control. Results are expressed as the mean relative absorbance (+s.d. of the population) of three replicates. ( e ) Rif R mutation profile of E. coli expressed WT A3G-CD2 and A3G-CD2 ‘YYFW’. Histogram showing the percent total mutation on specific rpoB nucleotide sequences. Results are expressed as the percentage of total mutations from six independent experiments with at least 20 colonies sequenced. Full size image To study the roles of each residue in the putative ssDNA-binding groove, alanine-mutants were generated for each position and characterized by BLI and ELISA. These two techniques allow cross-validation of the results and determination of equilibrium binding constants. ELISA studies showed that alanine substitutions at positions 277, 305, 307, 308, 309, 310, 313, 314, 367 and 369 resulted in reduced affinity for ssDNA ( Fig. 3d , Table 2 and Supplementary Fig. S2 ). Kinetic measurements with BLI revealed that alanine substitutions at W277, Y307, D313, K367 and Q369 resulted in the greatest decrease in affinity. Given the importance of W277 and Y307 in coordination of the target deoxycytidine, mutations to these residues, not surprisingly, displayed the largest decreases in ssDNA binding. Mutations distal to the active site (Y308A, F309A, W310A and Y314A) revealed smaller effects on ssDNA binding. The stability of each mutant was also assessed by circular dichroism (CD) spectroscopy (results presented in Supplementary Information ). In summary, mutations in the ssDNA-binding site did not affect the overall structure of A3Fc-CD2. Table 2 A3Fc-CD2 ssDNA-binding site mutations. Full size table Implication of an aromatic switch for substrate specificity In the A3Fc-CD2 structure, a series of aromatic residues in loop 7 (Y307, Y308, F309 and W310) line one side of the ssDNA-binding groove and are in the vicinity of the active site ( Fig. 3b ). Residues in A3Fc-CD2 loop 7 (Y307, Y308, F309 and W310) are capable of forming favourable stacking interactions with the nucleotide bases at positions −1 and −2 in A3F 5′- TT CA-3′ sequence element. Equivalent residues in A3A were shown by molecular docking studies to be involved in such interactions with the two nucleotides preceding the target cytidine [20] . These aromatic residues are not conserved across the A3 family ( Fig. 2c ), thus we predict that differences here may determine target DNA specificity. In A3F-CD2, this region is aromatic-rich, with a ‘YYFW’ motif (termed the nucleotide specificity box). However, in A3C and A3G-CD2, the ‘YYFW’ motif is replaced by ‘YYFQ’ and ‘YDDQ’ motifs, respectively. We propose that this ‘aromatic switch’ in the nucleotide specificity box determines substrate specificities in A3s. To test our hypothesis, we employed a heterologous bacterial DNA cytosine deaminase assay [18] to determine whether we are able to switch the substrate preference of A3G to A3F. The rpoB gene contains multiple mutable cytosines in various nucleotide sequence contexts. Thus, identification of rpoB mutational hotspots allows us to analyse substrate preferences at the nucleotide level. In agreement with previous studies, wild-type A3G-CD2 has a strong preference for 5′-C C -3′ dinucleotides ( Fig. 3e ) [18] , [30] , [31] . Mutating the ‘YDDQ’ nucleotide specificity box in A3G-CD2 to the aromatic-rich ‘YYFW’ counterpart in A3F-CD2 resulted in a complete change in substrate preference from 5′-C C -3′ to 5′-T C -3′ or 5′-G C -3′, suggesting four residues within the nucleotide specificity box is all that is necessary to confer substrate specificity ( Fig. 3e ). Moreover, the rpoB hotspots in A3G-CD2 ‘YYFW’ are in excellent agreement with those preferred by A3F. A direct HIV-1 Vif-A3F binding assay The analysis of A3 proteins to HIV-1 Vif have largely been limited to cell-based biochemical assays. To our knowledge, we have now developed the first direct in vitro binding assay, using BLI to measure the binding kinetics between full-length HIV-1 Vif and A3Fc-CD2. HIV-1 Vif is expressed in E. coli and refolded from inclusion bodies ( Supplementary Fig. S3A ). Refolded HIV-1 Vif was soluble and stable at low concentrations (<0.1 mg ml −1 ). A CD wavelength scan of the refolded Vif revealed a β-character protein ( Supplementary Fig. S3B ), consistent with previous studies [32] . A3Fc-CD2 bound to biotinylated full-length HIV-1 Vif with a dissociation equilibrium constant ( K d ) of 1.1 μM ( Supplementary Fig. S4 ). Our Vif-binding assay enabled us to map the HIV-1 Vif-binding interface at single-residue resolution, and provides a foundation for the development of new high-throughput assays. HIV-1 Vif-binding sites in A3Fc-CD2 Sequence analysis of HIV-1 Vif reveals a unique molecule with an abundance of positively charged (predicted pI>10) and hydrophobic residues. Previous studies have shown that a number of positively charged and hydrophobic motifs on HIV-1 Vif ( 11 Wx 2 SLVK 26 , 14 DRMR 17 , 55 VxIPLx 4 L 64 , 69 YxxL 72 , 74 TGERxW 79 , 81 LGxGx 2 IxW 89 , 96 TQx 5 ADx 2 I 107 and 171 EDRW 174 ) are involved in binding to A3F [17] , [33] , [34] , [35] , [36] . Therefore, a complementary binding surface on A3F-CD2 would be negatively charged and hydrophobic. Structural analysis of A3Fc-CD2 revealed a large negatively charged surface formed by the α3 and α4 helices, which is also conserved in A3C and A3D-CD2. Two negatively charged residues, E289 and E324, were previously identified to be involved in Vif binding [16] , [24] , [37] . However, the α3 and α4 helices also have a rich clustering of negatively charged residues (E286, E289, E316, S320 and E324) that we hypothesize to be important to Vif interaction ( Fig. 4 ). Substitution of any of these residues to alanine or glutamine completely abolished binding of A3Fc-CD2 to HIV-1 Vif ( Table 3 ). Mutation to a neighbouring arginine residue (R319A) had only minor effects on Vif binding, suggesting that only negatively charged or polar residues are directly involved in Vif binding. 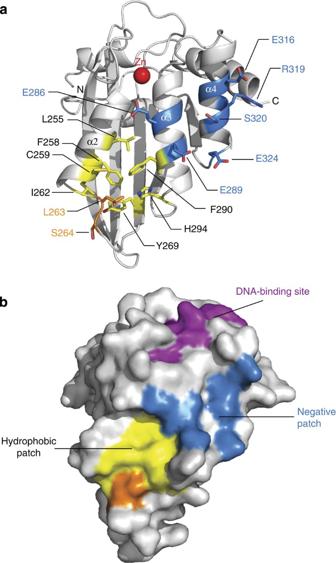Figure 4: A3Fc-CD2 HIV-1 Vif-binding site. (a) BLI kinetic analysis of A3Fc-CD2 binding to refolded full-length HIV-1 Vif. Biotin-labelled HIV-1 Vif was coupled to streptavidin-coated biosensors and monitored for binding to purified A3Fc-CD2 at 0, 0.4, 1, 2 and 4 μM concentrations. The data were analysed based on a 1:1 binding model, as only one A3F deamination motif is found on the ssDNA. The calculated fitted curves are shown as grey lines. (b) Putative Vif-binding residues. A number of aromatic and hydrophobic residues, coloured in yellow, (L255, F258, L263, Y269 and F290) are buried at the A3Fc-CD2 core. Residues L263 and S264 (shown in orange) were identified in this study to be not important for Vif binding. Figure 4: A3Fc-CD2 HIV-1 Vif-binding site. ( a ) BLI kinetic analysis of A3Fc-CD2 binding to refolded full-length HIV-1 Vif. Biotin-labelled HIV-1 Vif was coupled to streptavidin-coated biosensors and monitored for binding to purified A3Fc-CD2 at 0, 0.4, 1, 2 and 4 μM concentrations. The data were analysed based on a 1:1 binding model, as only one A3F deamination motif is found on the ssDNA. The calculated fitted curves are shown as grey lines. ( b ) Putative Vif-binding residues. A number of aromatic and hydrophobic residues, coloured in yellow, (L255, F258, L263, Y269 and F290) are buried at the A3Fc-CD2 core. Residues L263 and S264 (shown in orange) were identified in this study to be not important for Vif binding. Full size image Table 3 A3Fc-CD2 Vif-binding site mutations. Full size table Recent biochemical studies suggested that a hydrophobic V-shaped groove formed by the α2 and α3 helices of A3F participates in Vif binding [17] , [24] , [37] . This putative hydrophobic Vif-binding site is composed of residues L255, F258, C259, I262, L263, S264, Y269, F290 and H294 ( Fig. 4a,b ). To characterize the role of these hydrophobic residues, alanine- or charge-introducing (aspartate or lysine) mutations were generated. Using our BLI assay, we showed that mutations to L255, F258, C259, I262, Y269, F290 and H294 resulted in loss of Vif binding ( Table 3 ), consistent with previous biochemical studies [24] . However, the L263A and S264D mutations, which were previously shown to confer 100% resistance to Vif (ref. 24 ), resulted in K d values similar to wild-type A3Fc-CD2, questioning the importance of L263 and S264 in Vif binding ( Table 3 and Supplementary Fig. S4 ). The acquired immunodeficiency syndrome that results from HIV-1 infection remains a global health threat. Interactions between host restriction factors and viral antagonists, such as APOBEC3 and Vif, respectively, represent intriguing targets for the development of drugs to restrict viral replication and dissemination. In this study, we present the crystal structure of a chimeric A3F C-terminal domain containing the Vif-interaction interface. Our combinatorial approach encompassing structural, biochemical and biophysical studies provides insights into the molecular determinants of ssDNA binding, substrate specificity and, importantly, HIV-1 Vif binding. How the A3 proteins recognize single-stranded nucleic acids has been a controversial question. Structures of A3G-CD2 from NMR and X-ray crystallographic studies yielded at least two distinct models of ssDNA binding ( Fig. 3c ) [21] , [22] , [23] . Based on NMR data, Furukawa et al . [22] and Chen et al . [21] proposed that the DNA-binding site forms a straight groove, with loops 1 and 3 forming one side of the groove and loops 5 and 7 on the other (straight model). The crystal structure of A3G-CD2 and mutational data suggest an alternative mode of ssDNA binding, where the nucleic acid resides in a kinked groove (kinked model) [23] . In the kinked model, DNA contacts made through residues R213, H216, N244, Y315, D316, D317, Q318, R320, R374, R376 and W285 are proposed to create a bend in the groove ( Fig. 3c ). In A3Fc-CD2, the direction of the ssDNA-binding groove is most consistent with the ‘straight model’ of DNA binding ( Fig. 3c ). There are no grooves on the surface of A3Fc-CD2 that correspond to the A3G kinked channel. Detailed comparison of the A3Fc-CD2 and A3G-CD2 crystal structures reveals conformational differences in loops 1 and 7. In A3Fc-CD2, residues W209 and W310 in loops 1 and 7, respectively, appear to block the entrance of the kinked DNA channel. Mutations to residues along the A3F-CD2 straight ssDNA-binding groove (W277, R305, Y307, Y308, F309, W310 and Y314) confirm their importance in ssDNA binding. Interestingly, mutations in A3Fc-CD2 that are equivalent to residues proposed to contact ssDNA according to the A3G kinked model (D313, K367 and Q369) also resulted in a significant decrease in ssDNA binding ( Fig. 3d and Table 2 ). While our apo A3Fc-CD2 structure clearly shows a straight ssDNA-binding groove, a substrate-induced conformational change may bring these residues into proximity to bind ssDNA. In addition, it should be emphasized that our current structural understanding of A3 proteins is limited to the analysis of a single domain of A3 proteins. It may also be possible that ssDNA binds to residues identified in both the ‘straight’ and ‘kinked’ models of DNA binding in the context of full-length or higher-ordered oligomeric A3 protein structures. The A3 cytosine deaminase domains adopt similar structures; however, each has distinct substrate preferences. A3F-CD2 deaminates DNA cytosine within a 5′-T C -3′ sequence, whereas A3G recognizes 5′-C C -3′ (ref. 38 ). A3A and A3C target both 5′-T C -3′ and 5′-C C -3′ dinucleotides [20] , [39] . Our results suggest that the ‘YDDQ’ nucleotide specificity box in A3G-CD2 confers specificity for 5′-C C -3′ dinucleotides, whereas the ‘YYFW’ box in A3Fc-CD2 targets both 5′-T C -3′ and 5′-G C -3′ motifs. There is a clear trend; as the nucleotide specificity box motif becomes more negatively charged and polar, there is an increased preference for cytosine bases. This is consistent with the physiochemical differences between cytosine and thymine/guanine. The cytosine base is three times more hydrophilic than thymine [40] . The 4-amino group on the cytosine base can form hydrogen bonds to the aspartate or glutamine acceptors found in the A3G-CD2 ‘YDDQ’ nucleotide specificity box. An aromatic-rich ‘YYFW’ nucleotide specificity box in A3F-CD2 provides a more complementary environment for the hydrophobic thymidine nucleotides. A3C, which has only one glutamine in its ‘YYFQ’ nucleotide specificity box, recognizes a degenerate sequence—it is able to accommodate the substrates of both A3F (5′-T C -3′) and A3G (5′-C C -3′) [39] . Our study clearly demonstrates the importance of four residues in the nucleotide specificity box and a switch in hydrophobicities in determining substrate specificities in A3 proteins. Our current crystal structure and biophysical characterization of A3Fc-CD2 has revealed key determinants of Vif binding. The A3Fc-CD2 Vif-binding interface forms a shallow amphipathic cavity composed of residues from three helices (α2, α3 and α4 helix). Based on our Vif–A3F interaction assay, hydrophobic residues (L255, F258, C259, I262, Y269, F290 and H294) and negatively charged amino acids (E286, E289, E316 and E324) in A3Fc-CD2 were shown to be directly involved in Vif binding. However, solvent accessibility calculations revealed that residues in the hydrophobic Vif-binding groove, L255, F258, I262, Y269 and F290, have a side chain exposed surface area of <20% relative to random coil, suggesting that these residues are buried in the protein core and have a role in maintaining structural integrity. Alanine mutations in many of the hydrophobic residues affected the relative contents of secondary structural elements, as determined by CD spectroscopy (Supplementary Discussion and Supplementary Fig. S5 ), and resulted in a significant decrease in overall protein expression levels ( Table 3 ). In contrast, the mutations in the negatively charged residues did not affect expression levels and CD wavelength scans were superimposable ( Supplementary Fig. S6 ), suggesting no effects on overall structural stability. We suggest that the hydrophobic site is involved in maintaining the structural integrity and stability of A3Fc-CD2. However, it may be possible that the hydrophobic Vif-binding site has a role in both protein stability and Vif binding. Full characterization of the role of the hydrophobic site in Vif binding awaits the structural determination of an A3–Vif complex. The negatively charged Vif-binding site identified in this study now presents an attractive surface for the development of novel inhibitors capable of disrupting the A3-Vif interface. This negatively charged Vif-binding site is well conserved in A3C and a homology model of A3D-CD2 ( Fig. 5 ), suggesting a common mode of Vif binding for the A3F-CD2 Z2-type DNA cytosine deaminase domains. While the Vif-binding A3G-CD1 domain also belongs to the Z2-class of DNA cytosine deaminase domains, it shares only 43% sequence identity with A3F-CD2 and the residues implicated in Vif binding are not conserved. The electrostatic potential surface of A3G-CD1 reveals a replacement of the negatively charged patch in A3Fc-CD2 with a positively charged surface ( Fig. 5 ). Moreover, a ‘DPD’ motif in loop 7 of A3G-CD1 previously implicated in Vif binding [41] does not overlap with the negatively charged surfaces in A3F-CD2, A3C and A3D-CD2. This suggests that A3G-CD1 adopts a unique Vif-binding interface that is distinct from other A3F-like Z2-cytosine deaminase domains. The electrostatic surface of A3H, a Z3-DNA cytosine deaminase, is different from all other A3 proteins ( Fig. 5 ). Based on the current A3 structural models, there are likely multiple A3 interfaces that can interact with Vif. 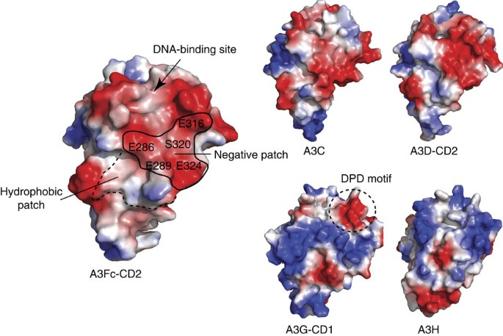Figure 5: Surface electrostatic potential of APOBEC3 proteins. A negatively charged surface conserved with other Z2-cytosine deaminase domains is proposed to be important for Vif-binding. Electrostatic potential mapped onto the molecular surface of A3C (PDB: 3VOW), and the homology models of A3D-CD2, A3G-CD1 and A3H. The proposed footprints of the A3 negative and hydrophobic patch involved in Vif binding are shown by the solid and dashed lines, respectively. A previously characterized ‘DPD’ motif involved in A3G Vif binding is displayed for the A3G-CD1 homology model. Red and blue coloured regions denote negative and positive charges, respectively. Note: the ssDNA-binding site is at the top of the depicted A3 molecules and has no overlap with the hydrophobic or negatively charged Vif-binding site. Figure 5: Surface electrostatic potential of APOBEC3 proteins. A negatively charged surface conserved with other Z2-cytosine deaminase domains is proposed to be important for Vif-binding. Electrostatic potential mapped onto the molecular surface of A3C (PDB: 3VOW), and the homology models of A3D-CD2, A3G-CD1 and A3H. The proposed footprints of the A3 negative and hydrophobic patch involved in Vif binding are shown by the solid and dashed lines, respectively. A previously characterized ‘DPD’ motif involved in A3G Vif binding is displayed for the A3G-CD1 homology model. Red and blue coloured regions denote negative and positive charges, respectively. Note: the ssDNA-binding site is at the top of the depicted A3 molecules and has no overlap with the hydrophobic or negatively charged Vif-binding site. Full size image Our crystal structure presented in this manuscript has now identified well-defined sites on A3Fc-CD2 involved in ssDNA and Vif binding. We have also identified novel structural determinants that explain the differences in substrate specificities between A3 family members. Collectively, our studies and findings will be invaluable to the A3 community by providing the relevant structural scaffold for the development of effective HIV-1 inhibitors aimed at selectively disrupting the A3F-Vif interface. Footnote: while this manuscript was under review, structures of A3A [20] and a C-terminal domain of A3F [42] (with 11 amino-acid substitutions required for solubilization, termed A3F 11X -CD2) were reported. The structures of A3A and A3F 11X -CD2 align well with A3Fc-CD2. Interestingly, no conformational changes in the chimeric region of A3Fc-CD2 exist. Expression and purification of APOBEC3F The DNA corresponding to A3F (residues 218–373) with an A3G solubilization linker (residues 197–221) at the N terminus was codon-optimized and whole-gene-synthesized (Biobasic Inc). This A3Fc-CD2 gene was subsequently cloned, according to manufacturer’s protocol, into a pET46-Ek/LIC vector (EMD Millipore) containing an N-terminal His-tag, and thrombin and TEV cleavage sites ( Supplementary Fig. S1 ). A3Fc-CD2 and mutants were expressed in Rosetta-2 (DE3) E. coli cells. Cell cultures were grown to OD 600 =0.8 and induced with a final concentration of 0.5 mM IPTG for 18 h at 25 °C. Cells were resuspended in Ni-binding buffer (50 mM Tris-HCl pH 8.0, 300 mM NaCl and 20 mM imidazole) with EDTA-free protease inhibitor cocktail and lysed at 30 kpsi using a hydraulic cell disruption system (Constant Systems TS benchtop). The lysate was centrifuged to remove cellular debris prior to loading onto Ni-NTA resin (Thermo Pierce). A3Fc-CD2 was washed with Ni-NTA binding buffer with 50 mM imidazole. A3Fc-CD2 was eluted by a two-step gradient of Ni-binding buffer with 125 mM imidazole and Ni-binding buffer with 500 mM imidazole. Fractions that contained A3Fc-CD2 were concentrated and purified on a Superdex-200 10/300 GL column equilibrated in Buffer A (10 mM Tris-HCl pH 7.5, 0.3 M NaCl, 0.05% ( w / v ) CHAPS and 2 mM TCEP). For structural studies, A3Fc-CD2 was further purified by anion exchange chromatography. Here A3Fc-CD2 was pooled and loaded onto a MonoQ HR 5/5 column equilibrated in Buffer B (10 mM Tris-HCl pH 7.5, 0.1 M NaCl, 0.05% ( w / v ) CHAPS and 2 mM TCEP). A3Fc-CD2 was eluted using a linear gradient of 0–100% Buffer B with 1 M NaCl. Purified A3Fc-CD2 was quantified by A 280 and concentrated to 20 mg ml −1 for crystallization. Crystallization and data collection Initial crystals were obtained by mixing a 1:1 ratio of A3Fc-CD2 protein and 18% ( w / v ) PEG 8000, 0.1 M CHES pH 9.0 and 25% ( w / v ) glucose on a cover slide and equilibrating over a reservoir of 20% ( w / v ) PEG 8000 and 0.1 M CHES pH 9.0 for 10 min. Subsequently, the cover slide was transferred over to a reservoir containing 18% ( w / v ) PEG 8000, 0.1 M CHES pH 9.0 and 25% ( w / v ) glucose, and allowed to grow at 20 °C. Needle-like crystals appeared over a 5-day period and were crushed using a glass pedestal. Random matrix microseeding [43] was performed using a Douglas Instruments Oryx 8 to obtain additional crystallization hits. High-quality crystals were obtained by mixing a 3:1 ratio of A3Fc-CD2 protein to seed stock, and equilibrating over a reservoir of 0.17 M magnesium formate, 20% ( v / v ) glycerol and 10% ( w / v ) glucose. Wedge-like crystals were harvested and directly flash-cooled in liquid nitrogen. A complete data set was collected at the Advanced Photon Source (Argonne National Laboratories, Argonne, IL, USA), Beamline 24-ID-E. Data were indexed, integrated and scaled using d*trek [44] . Structural determination The A3Fc-CD2 structure was determined by molecular replacement, using the programme Phaser [45] and the A3C structure (PDB code: 3VOW) [24] as the search model. Two clear solutions were identified. Iterative rounds of model rebuilding and simulated annealing torsion angle refinement were performed using the programme Coot [46] and PHENIX.refine [47] . Identification of proper sequence registry was confirmed with the location of the catalytic zinc site and the presence of bulky aromatic residues. Molprobity [48] was used throughout the refinement to ensure that clashes, rotamers, Asn/Gln/His flips and Ramachandran outliers were minimized. Ramachandran plot analysis revealed that 97.2 and 2.8% of residues are in favored and disallowed regions, respectively. Residues in disallowed regions reside in regions with weaker electron density. The final model contains A3F residues 218–373 and A3G residues 197–219. Weak electron density was observed for residues 225–236. Homology models were generated using the Phyre2 Protein Fold Recognition Server [49] . All molecular ribbon diagrams and vacuum electrostatic calculations were generated using the programme MacPyMOL. BLI DNA–protein interaction studies The binding of ssDNA (5′-TCCCTCAGACCCTTTTAGTCAGTGTGGAAAATCTCTAGCAGT-3′) to A3Fc-CD2 was measured by BLI using a BLItz instrument (Pall/ForteBio). The sequence corresponds to the viral U5 end of the 3′-LTR and was shown to bind to A3F [50] . This ssDNA has one A3F deamination site (5′-CT C A-3′). Biotinylated ssDNA was diluted to 50 μM in kinetics buffer (PBS, 0.1% ( w / v ) BSA, and 0.002% ( v / v ) Tween-20), immobilized on a streptavidin biosensor for 120 s. For the A3Fc-CD2 mutants, 20 μM of biotinylated ssDNA was immobilized on the probe. A3Fc-CD2 was diluted into kinetics buffer (0, 0.4, 1, 2 and 4 μM) and association to the biotinylated ssDNA was measured over 300 s. Subsequently, the biosensor was immersed in kinetics buffer for 300 s to measure dissociation. The K d was calculated using the BLItz Pro v.1.1.0.28 software. DNA–protein interaction ELISAs Single-stranded 42-mer DNA ( Fig. 1c ) was synthesized (Integrated DNA Technologies). Biotinylated ssDNA (1.5 pmol) was immobilized onto a streptavidin-coated ELISA plate (Quidel) and washed three times with PBS with 0.01% ( v / v ) Tween-20 (PBS-T). Wells were blocked with 3% ( w / v ) BSA in PBS-T overnight at 4 °C. 25, 50, 75 and 100 μg of A3Fc-CD2 or A3Fc-CD2 mutants were incubated at 22 °C for 1.5 h and subsequently washed three times with PBS-T. A mouse anti-His primary mAb (Roche) diluted 1:3,000 in PBS-T was incubated for 1 h at 22 °C. The plate was washed three times prior to incubation with a goat anti-mouse HRP-conjugated secondary mAb (Pierce) diluted 1:3,000. The plates were developed using TMB-One substrate solution (Kem-En-Tec Diagnostics) for 5 min. Colour development was stopped with 2 N sulphuric acid and measured at 495 nm. As a negative control, the biotinylated sense and antisense DNA strands (3′-AGG GAG TCT GGG AAA ATC AGT CAC ACC TTT TAG AGA TCG TCA-5′) were heated at 95 °C for 15 min and allowed to cool to 22 °C in annealing buffer (10 mM Tris-HCl (pH 7.5), 1 mM EDTA and 50 mM NaCl). The double-stranded DNA probe was then immobilized onto the streptavidin-coated ELISA plate and performed as described above. All experiments were performed in triplicate. Bacterial cytosine deaminase assay A bacterial E. coli based rifampicin resistant (Rif R ) mutation assay was used to monitor the degree of DNA cytosine deaminase activity [18] . Wild-type A3G-CD2 (residues 197–384), A3G-CD2 ‘YYFW’, A3Fc-CD2 or A3Fc-CD2 ssDNA-binding mutants cloned into pET46-Ek/LIC were transformed into BL21-(DE3) E. coli cells. Single colonies were used to inoculate a 10 ml culture of LB supplemented with 100 μg ml −1 ampicillin. At OD 600 =0.6, the cultures were induced with 1 mM final concentration of IPTG and grown overnight at 37 °C. Cell cultures were normalized (7 ml of cells at OD 600 =0.5) and plated onto LB-agar plates containing 100 μg ml −1 rifampicin to select for Rif R clones. Single colonies were picked from plates and colony PCR was performed to amplify the bacterial RNA polymerase gene rpoB . The rpoB PCR products were DNA sequenced with an rpoB sequencing primer (5′-GGC-GAA-ATG-GCG-GAA-AAC-3′). A3F or A3G DNA-binding motifs in the rpoB gene were analysed for C–to-T mutations. CD and thermal melts CD wavelength scans and thermal titrations were performed on all A3Fc-CD2 proteins at a concentration of 1.0 mg ml −1 in PBS, 0.05% ( w / v ) CHAPS and 1 M guanidine-HCl on a Jasco J-810 spectropolarimeter. CD wavelength scans collected between 190–250 nm using a 1-mm quartz cuvette (Helma) were averaged over five scans. Thermal denaturation of A3Fc-CD2 and mutants were performed by increasing the temperature from 20–95 °C and monitoring the loss in CD signal at 222 nm. BLI Vif-APOBEC3F interaction studies HIV-1 Vif was expressed in BL21-(DE3) E. coli cells, purified and refolded from inclusion bodies, as previously described [32] . Briefly, Vif inclusion bodies were resolubilized in 6 M guanidine–HCl and 10 mM Tris–HCl (pH 7.4) overnight at 22 °C, and subsequently clarified by centrifugation prior to Ni-NTA purification. The Ni-NTA column was washed with 8 M urea, 100 mM NaH 2 PO 4 and 10 mM Tris-HCl (pH 6.9), and Vif was eluted in the same buffer at pH 4.5. Vif was subsequently purified on a prep grade Superdex-75 10/300 column equilibrated in 8 M urea, 100 mM NaH 2 PO 4 , 10 mM β-mercaptoethanol and 10 mM Tris-HCl pH 4.5. The peak corresponding to monomeric Vif was collected and diluted to 0.1 mg ml −1 and dialyzed against 100 mM NaH 2 PO 4 , 10 mM Tris-HCl, 150 mM NaCl, 20% ( v / v ) glycerol (pH 6.0) with decreasing concentration of urea (6, 4, 2, 1 and 0.5 M). The final refolded HIV-1 Vif was dialyzed against 10 mM NaH 2 PO 4 pH 6.0, 150 mM NaCl and 20% ( v / v ) glycerol, and biotinylated using the EZ-Link Sulfo-NHS-LC-Biotinylation kit (Thermo Pierce) according to the manufacturer’s protocol. Excess biotin was removed by dialysis. Biotinylated Vif was diluted to 40 μg ml −1 in 10 mM NaH 2 PO 4 , 150 mM NaCl, 20% ( v / v ) glycerol, 1 mg ml −1 BSA and 0.002% ( v / v ) Tween-20 and immobilized onto a BLI streptavidin probe for 120 s. A3Fc-CD2 mutants were diluted into 10 mM Tris-HCl (pH 7.5), 150 mM NaCl, 0.05% ( w / v ) CHAPS, 1 mg ml −1 BSA and 0.002% ( v / v ) Tween-20 and allowed to associate over 80 s. Dissociation was monitored over 110 s. Purified A3G-CD2 was used as a negative control. Accession codes: Atomic coordinates and structure factors for A3Fc-CD2 have been deposited in the Protein Data Bank (PDB) with the accession code 4J4J . How to cite this article: Siu, K. K. et al . Structural determinants of HIV-1 Vif susceptibility and DNA binding in APOBEC3F. Nat. Commun. 4:2593 doi: 10.1038/ncomms3593 (2013).